Structural basis for endotoxin neutralisation and anti-inflammatory activity of thrombin-derived C-terminal peptides Thrombin-derived C-terminal peptides (TCPs) of about 2 kDa are present in wounds, where they exert anti-endotoxic functions. Employing a combination of nuclear magnetic resonance spectroscopy (NMR), biophysical, mass spectrometry and cellular studies combined with in silico multiscale modelling, we here determine the bound conformation of HVF18 (HVFRLKKWIQKVIDQFGE), a TCP generated by neutrophil elastase, in complex with bacterial lipopolysaccharide (LPS) and define a previously undisclosed interaction between TCPs and human CD14. Further, we show that TCPs bind to the LPS-binding hydrophobic pocket of CD14 and identify the peptide region crucial for TCP interaction with LPS and CD14. Taken together, our results demonstrate the role of structural transitions in LPS complex formation and CD14 interaction, providing a molecular explanation for the previously observed therapeutic effects of TCPs in experimental models of bacterial sepsis and endotoxin shock. Lipopolysaccharide (LPS) sensing by Toll-like receptor 4 (TLR4) is crucial in early responses to infection, where an uncontrolled LPS response gives rise to excessive localised inflammation, such as that found in infected wounds, but also in severe systemic responses to infection [1] , [2] . Therefore, although sensing of LPS is important for initial host defence responses, clearance and control of this molecule is critical in order to avoid excessive inflammation and organ damage. For example, LPS triggers NF-κB-mediated upregulation of tissue factor, and thus formation of thrombin, which in turn activates coagulation and fibrin formation, thereby aiding in initial hemostasis and defence against bacterial invasion [3] . Furthermore, proteolysis of thrombin by neutrophil elastase leads to formation of aggregation-prone 11 kDa C-terminal fragments which are present in wounds, and form amorphous amyloid-like co-aggregates with both LPS and Gram-negative bacteria, aiding in the subsequent clearance of these aggregates by phagocytosis [4] . In addition, thrombin-derived C-terminal peptides (TCP) of roughly 2 kDa, such as FYT21 (FYTHVFRLKKWIQKVIDQFGE) and HVF18 (HVFRLKKWIQKVIDQFGE), are present in wound fluids [5] , [6] , and have been demonstrated to exert anti-endotoxic functions in vitro and in vivo [7] , [8] . Such smaller peptides belong to the diverse family of host-defence peptides (HDPs) [9] , which includes neutrophil-derived α-defensins and the cathelicidin LL-37 [10] , all known to exhibit immunomodulatory activities [11] . Today, there is an urgent need for novel anti-infective therapies [12] . However, current treatments based on antibiotics target bacteria only, and not the accompanying over-activation of immune responses. This uncontrolled stimulation may cause an overwhelming production of inflammatory cytokines leading to systemic inflammation, intravascular coagulation and organ dysfunction, such as seen in sepsis [13] . This is a leading cause of death in the US alone, with over 700,000 cases estimated every year, and with mortality rates from 28 to 60% [14] . Treatment concepts based on Nature’s own innate defence strategies, aiming at not only targeting bacteria, but also the excessive immune response, could therefore have a significant therapeutic potential. For instance, many naturally occurring HDPs, as well as fragments of LPS-recognising proteins, display a strong affinity for LPS, blocking downstream interaction with LPS-binding protein (LBP), thereby reducing cytokine production in vitro and in vivo [15] , [16] , [17] . Neutralisation of circulating LPS by HDPs has been shown to reduce adverse LPS-induced pro-inflammatory effects in experimental animal models [7] , [18] , [19] . In this context, a prototypic TCP, GKY25 (GKYGFYTHVFRLKKWIQKVIDQFGE), encompassing sequences of natural TCPs previously identified in human wounds [6] , has been shown to neutralise LPS in vitro and protect against P. aeruginosa sepsis and LPS-mediated shock in experimental animal models, mainly via reduction of systemic cytokine responses [7] , [8] , [20] . Hypothetically, it could be argued that mere LPS-binding, via scavenging, could explain the observed peptide effects. However, a TCP-variant (WFF25) with identical composition but a re-organised sequence, yielding a linear amphipathic structure with retained (and even higher) LPS-affinity [21] , displayed neither cell binding and uptake, nor any anti-endotoxic effects in vitro and in vivo despite its higher LPS and lipid A binding. Moreover, electron microscopy studies showed that TCPs co-localise with LPS on the monocyte cell surface, and subsequently internalise with LPS, without any concomitant TLR4 dimerisation and downstream NF-κB activation. Furthermore, pre-incubation with TCPs, followed by addition of LPS yielded similar effects, suggestive of a cell-dependent activity [20] . These observations hinted at the existence of additional targets for TCPs apart from LPS, in line with previous observations of structurally unspecific LPS binding not being a sufficient requirement of HDP anti-endotoxic effects [22] . With this background, we set out to characterise the structural prerequisites at the molecular level which underlie the anti-endotoxic actions of such TCPs. Here, employing NMR analysis, we determine the bound conformation of the TCP HVF18 in complex with LPS. The HVF18-LPS structure comprises a C-terminal helix and extended N-terminus with a β-turn that favours a curved backbone fold, imparting a C-shaped amphipathic arrangement of the hydrophobic core lined with two hydrophilic clusters. Moreover, using a combination of in silico docking, microscale thermophoresis (MST) analysis, and chemical crosslinking followed by mass spectrometry analyses, we show that that TCPs bind to the amino terminal hydrophobic LPS binding pocket of human CD14. In addition, we observe that the affinity of LPS for CD14 is reduced in the presence of TCPs, illustrating the competitive nature of TCP action. Taken together, we define TCP interactions with LPS and CD14 and provide a detailed explanation for the previously observed anti-endotoxic effects of TCPs in vitro and in vivo. Background of peptides studied The C-terminal region of thrombin, GKYGFYTHVFRLKKWIQKVIDQFGE, the sequence of which is highlighted in the crystal structure (shown in Fig. 1a ), comprises a flexible β-strand segment and a compact amphipathic helix. Previous studies have shown that various proteases can generate TCPs derived from this region [6] . For illustrative purposes, and to highlight the complete, albeit gradual, formation of such fragments, the generation of the 2 kDa TCP HVF18 (HVFRLKKWIQKVIDQFGE), cleaved out by human neutrophil elastase [8] , is depicted in Fig. 1b . A similar generation of the peptide FYT21 (FYTHVFRLKKWIQKVIDQFGE) has been observed with the bacterial M4 peptidases Pseudomonas aeruginosa elastase [5] , [6] and Staphylococcus aureus aureolysin [6] . The prototypic peptide GKY25 (GKYGFYTHVFRLKKWIQKVIDQFGE), incorporating these endogenous sequences, has been further used in in vitro studies on its mode-of-action, as well as in several therapeutic in vivo studies, aimed at targeting endotoxin-mediated inflammatory responses [7] , [8] . The truncated peptide variant VFR12 (VFRLKKWIQKVI) has been shown to constitute a minimal LPS binding site while not exhibiting any anti-endotoxic effects in cell models [23] . Some key physicochemical parameters of these TCPs are indicated in Fig. 1c . Fig. 1 Thrombin C-terminal peptides, and their binding to E. coli LPS. a 3D model of human α-thrombin (PDB code 1C5L) highlighting thrombin C-terminal peptide fragment. b Western blot analysis of human α-thrombin incubated with neutrophil elastase (NE) for the indicated time period generates thrombin C-terminal peptide fragments of varying lengths. The synthetic peptide HVF18 is loaded as molecular size control corresponding to generated fragments. The marker lane is from the same blot but aligned for clarity. c Table showing thrombin C-terminal peptides amino acid sequences and physicochemical properties determined using Heliquest online server tool. The hydrophobicity and amphipathicity of VFR12 was too short for accurate determination using Heliquest. d Representative intrinsic tryptophan fluorescence emission spectra of HVF18 titrated with increasing concentration of E. coli LPS. e LPS binding affinity of peptides determined from changes in emission maxima ( λ max ) upon titration, fitted with Graph Pad Prism v7.02 one-site binding model. Results are means ± SD of three experiments. f Ellipsometry showing peptide binding to E. coli LPS preabsorbed on solid supports. Results are means ± SD of two experiments. g Representative kinetic curves showing corresponding peptide adsorption. All experiments were performed in 10 mM Tris, pH 7.4 Full size image Interaction of TCPs with LPS Intrinsic tryptophan fluorescence was employed to monitor the interaction of the TCPs with E. coli LPS. 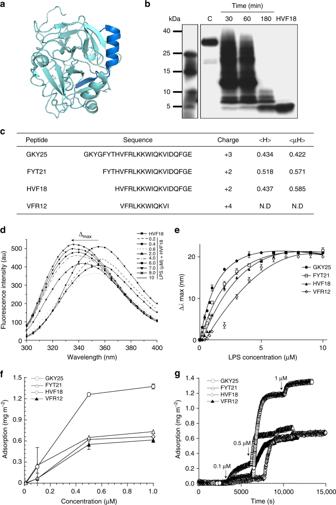Fig. 1 Thrombin C-terminal peptides, and their binding toE. coliLPS.a3D model of human α-thrombin (PDB code 1C5L) highlighting thrombin C-terminal peptide fragment.bWestern blot analysis of human α-thrombin incubated with neutrophil elastase (NE) for the indicated time period generates thrombin C-terminal peptide fragments of varying lengths. The synthetic peptide HVF18 is loaded as molecular size control corresponding to generated fragments. The marker lane is from the same blot but aligned for clarity.cTable showing thrombin C-terminal peptides amino acid sequences and physicochemical properties determined using Heliquest online server tool. The hydrophobicity and amphipathicity of VFR12 was too short for accurate determination using Heliquest.dRepresentative intrinsic tryptophan fluorescence emission spectra of HVF18 titrated with increasing concentration ofE. coliLPS.eLPS binding affinity of peptides determined from changes in emission maxima (λmax) upon titration, fitted with Graph Pad Prism v7.02 one-site binding model. Results are means ± SD of three experiments.fEllipsometry showing peptide binding toE. coliLPS preabsorbed on solid supports. Results are means ± SD of two experiments.gRepresentative kinetic curves showing corresponding peptide adsorption. All experiments were performed in 10 mM Tris, pH 7.4 Figure 1d shows changes in the fluorescence emission spectra of HVF18 as a function of LPS concentration. In the absence of LPS, the tryptophan residue has an emission maximum at 357 nm. Addition of LPS results in a concentration-dependent blue shift in the emission maximum, indicating peptide binding to LPS. A similar shift in emission maximum was observed for the other TCPs, although differences in the extent of the blue shift were noted (Supplementary Figure 1 ). The change in fluorescence emission maxima ( λ max ) of the TCPs was utilised to obtain an indication of peptide binding affinities to LPS (Fig. 1e ). As shown in Supplementary Table 1 , GKY25 displayed the highest affinity ( K d = 2 ± 0.29 μM) among the peptides investigated, followed by the endogenous fragments HVF18 ( K d = 4.24 ± 0.90 μM), and the shorter VFR12 ( K d = 11.45 ± 0.45 μM). Furthermore, the localisation of the tryptophan residue in the LPS complexes was determined by quenching of the tryptophan fluorescence with a neutral quencher, acrylamide. Supplementary Table 1 shows the obtained Stern-Volmer quenching constants ( K SV ) of the peptide in unbound and LPS-boundstates. Although many factors determine the photophysics of tryptophan, a large K SV for the peptides in their unbound state generally indicates complete exposure of the tryptophan residue to buffer, while a low K SV in the LPS-bound states implicates that exposure of the tryptophan to the solvent is restricted owing to incorporation of the tryptophan side chain into the hydrophobic milieu of LPS. By analogy, ellipsometry results indicate that TCPs bind substantially to LPS. GKY25 adsorbed to LPS with the highest affinity among the peptides investigated, followed by FYT21, HVF18, and VFR12 (Fig. 1f ). Thus, at increasing peptide concentrations, peptide length affects LPS binding, indicating the importance of hydrophobic interactions required for LPS penetration (Fig. 1f ). The kinetics of peptide binding is also exemplified (Fig. 1g ). Taken together, the ellipsometry and tryptophan fluorescence results indicate that TCPs bind LPS. Neutralisation of LPS by TCPs Next, we assessed the ability of the peptides to neutralise LPS in solution using the highly sensitive limulus amebocyte lysate (LAL) assay. As can be seen in Fig. 2a , GKY25, FYT21, and HVF18, but not VFR12, neutralised LPS in the LAL assay in the dose range studied, and a length-dependent inhibitory activity was observed, corresponding to the ellipsometry and tryptophan fluorescence data outlined above. Likewise, using LPS-stimulated THP-1 monocytes and evaluation of NF-κB activation, a similar blocking of endotoxin responses was observed (Fig. 2b ), in which VFR12 did not block NF-κB activation (Supplementary Figure 1d ). Notably, the peptide FYT21, previously identified in infected wounds [5] , [6] , blocked LPS-induced pro-inflammatory response and displayed LPS neutralisation to a similar extent as GKY25, previously used in therapeutic studies (Fig. 2b ). Also notable is that the fragments FYT21 and HVF18 share relevant physiological concentrations for both thrombin and other TCPs [4] . Overall, these data demonstrate TCPs ability to neutralise LPS and block LPS-induced pro-inflammatory responses in vitro. Fig. 2 Thrombin C-terminal peptides bind and inhibit LPS-induced proinflammatory responses. a Limulus amebocyte lysate (LAL) chromogenic assay showing variations in TCPs ability to neutralise E. coli LPS in solution. Results are means ± SD of two experiments. b Inhibition of NF-kB activation in THP-1 monocytes stimulated with 10 ng ml −1 E. coli LPS upon treatment with indicated TCPs at the specified concentrations, 20 h post stimulation. Results are means ± SD of at least six experiments Full size image NMR studies of TCPs in free and LPS-bound states NMR structural studies were employed to gain further insight into the molecular interactions of TCP-LPS complex formation. 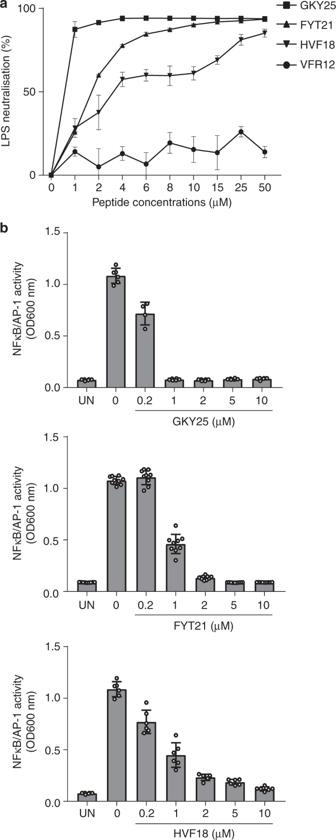Fig. 2 Thrombin C-terminal peptides bind and inhibit LPS-induced proinflammatory responses.aLimulus amebocyte lysate (LAL) chromogenic assay showing variations in TCPs ability to neutraliseE. coliLPS in solution. Results are means ± SD of two experiments.bInhibition of NF-kB activation in THP-1 monocytes stimulated with 10 ng ml−1E. coliLPS upon treatment with indicated TCPs at the specified concentrations, 20 h post stimulation. Results are means ± SD of at least six experiments The spin systems in the TOCSY spectra of VFR12 and HVF18 are well dispersed and permit complete assignment of proton resonances (Supplementary Figure 2a, b ). However, in the case of FYT21 and GKY25, the N-terminal (GKYGFYTHV) proton resonances overlapped or were absent, rendering assignment incomplete (Supplementary Figure 2c, d ). Changes in D 2 O (5%) and pH did not improve the spin system assignments. Nonetheless, the NOESY spectra of the free peptides were largely characterised by weak intra-residue (CαH i /NH i ) and sequential (CαH i /NH i+ 1 ) connectivities between backbone proton resonances (Supplementary Figure 2 ). The absence of medium- ( i to i + 2/ i + 3/ i + 4) and long-range nuclear Overhauser enhancements (NOEs), particularly involving aromatic side-chain proton resonances (6.8–7.5 ppm) clearly indicate that the TCPs are highly dynamic in solution, consistent with the random coil observation from circular dichroism (CD) spectra (Supplementary Figure 2e ). 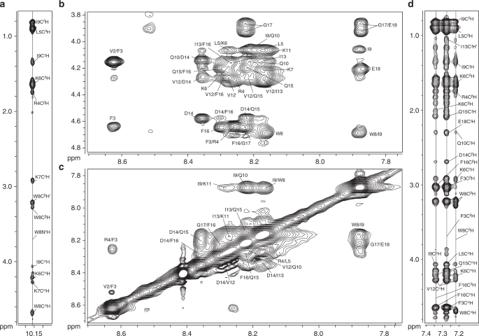Fig. 3 tr-NOESY spectrum of HVF18 in LPS micelles. Two-dimensional1H–1H tr-NOESY spectrum of HVF18 (0.5 mM) in the presence of LPS (20 μM) (a) showing NOE connectivities involving W8 indole proton with the upfield shifted aliphatic proton resonances.bFinger print region showing sequential and medium range NOE connectivities between backbone alpha and amide proton (CαH/HN) resonances, (c) section showing NOE connectivities among backbone amide (HN/HN) resonances and (d) section showing NOE connectivities between the aromatic ring protons of F3, F16, and W8 with the upfield shifted aliphatic proton resonances. tr-NOESY spectrum of HVF18 in LPS micelles was obtained in aqueous solution (pH 4.5) at 298 K in a Bruker DRX 600 MHz NMR instrument A series of 1D 1 H– 1 H spectra of GKY25 or FYT21 with successive addition of LPS showed prominent chemical shifts in proton resonances of the backbone and side-chain regions (Supplementary Figure 3a, b ). Moreover, visible aggregates formed, indicating that the peptides do not undergo fast-to-intermediate exchanges between free and LPS-bound states within the NMR time-frame, thus precluding three-dimensional structure determination. Nonetheless, in the case of HVF18 or VFR12, addition of LPS yielded concentration-dependent line broadening of the backbone and side-chain proton resonances without any significant chemical shift changes, enabling LPS-bound structure determination using tr-NOESY (Supplementary Figure 3c, d ). The tr-NOESY spectra of HVF18 showed a drastic improvement in the number and intensity of NOE cross-peaks, involving backbone and side-chain proton resonances in the presence of LPS (Fig. 3 ). The down-field shift of the indole proton of W8 (~10.17 ppm), as well as of the degenerate aromatic ring protons of Phe (7.35–7.25 ppm), showed several NOE connectivities with aliphatic side-chain proton resonances of residues L5, I9, V12, I13 (Fig. 3a, d ). Interestingly, NOEs involving the indole proton of W8 with the CαH and CβH of R4, K6, and K7 were also identified. Together, these results demonstrate conformational stabilisation and the occurrence of side-chain interactions in LPS-bound HVF18. Fig. 3 tr-NOESY spectrum of HVF18 in LPS micelles. Two-dimensional 1 H– 1 H tr-NOESY spectrum of HVF18 (0.5 mM) in the presence of LPS (20 μM) ( a ) showing NOE connectivities involving W8 indole proton with the upfield shifted aliphatic proton resonances. b Finger print region showing sequential and medium range NOE connectivities between backbone alpha and amide proton (CαH/HN) resonances, ( c ) section showing NOE connectivities among backbone amide (HN/HN) resonances and ( d ) section showing NOE connectivities between the aromatic ring protons of F3, F16, and W8 with the upfield shifted aliphatic proton resonances. 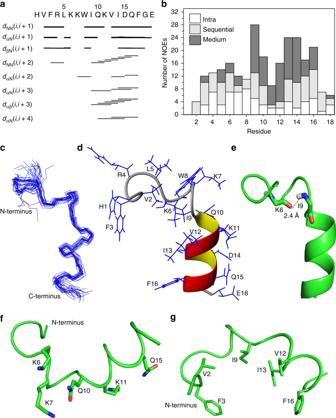Fig. 4 Analyses of tr-NOESY spectrum and three-dimensional solution structure of HVF18 in LPS micelles.aDiagram summarising the sequential and medium range NOE contacts identified in HVF18.bBar diagram showing number and type of NOEs observed for HVF18 in complex with LPS as a function of amino acids.cSuperposition of backbone atoms (N, Cα, C’) for the 20 lowest energy conformers of LPS-bound HVF18.dA representative structure of LPS-bound HVF18 showing backbone topology and side-chain dispositions and (e) plausible hydrogen bond formation between K6 and I9 in the β-turn region. Ribbon representation of peptide backbone showing amphipathic disposition of (f) hydrophilic residues along the convex side (g) and the hydrophobic residues on the concave side of a curved backbone fold of HVF18 in complex with LPS. Figures were generated using MolMol v2K.2 and Pymol v1.7.4.0 tr-NOESY spectrum of HVF18 in LPS micelles was obtained in aqueous solution (pH 4.5) at 298 K in a Bruker DRX 600 MHz NMR instrument Full size image Figure 4a summarises the tr-NOEs of HVF18 observed in the presence of LPS. Intense sequential (CαH i /NH i +1 ) , as well as backbone NH/NH, NOEs are seen for most residues, except for overlap of the CαH proton resonances with backbone amide proton resonances (ω2) for a few residues. Several medium-range NH/NH ( i to i + 2) NOEs and Cα/NH ( i to i + 2, i + 3 and i + 4) NOEs could be observed for the C-terminal region I9-G17 residues, suggesting an α-helical conformation. In contrast, the N-terminal region H1-W8 is characterised by the presence of strong sequential (CαH i /NH i +1 ) , NH/NH and a few NH/NH ( i, i + 2) NOEs, suggesting a lack of helical conformation at the amino terminus. Fig. 4 Analyses of tr-NOESY spectrum and three-dimensional solution structure of HVF18 in LPS micelles. a Diagram summarising the sequential and medium range NOE contacts identified in HVF18. b Bar diagram showing number and type of NOEs observed for HVF18 in complex with LPS as a function of amino acids. c Superposition of backbone atoms (N, Cα, C’) for the 20 lowest energy conformers of LPS-bound HVF18. d A representative structure of LPS-bound HVF18 showing backbone topology and side-chain dispositions and ( e ) plausible hydrogen bond formation between K6 and I9 in the β-turn region. Ribbon representation of peptide backbone showing amphipathic disposition of ( f ) hydrophilic residues along the convex side ( g ) and the hydrophobic residues on the concave side of a curved backbone fold of HVF18 in complex with LPS. Figures were generated using MolMol v2K.2 and Pymol v1.7.4.0 Full size image Likewise, for VFR12 a large number of intense NOE cross-peaks, involving backbone and side-chain proton resonances were observed in the presence of LPS (Supplementary Figure 4 ). As above, the continuity of sequential ( i to i + 1) NH/NH and Cα/NH NOEs was disturbed due to overlap. However, few medium-range ( i to i + 2) NH/NH NOEs and ( i to i + 2, i + 3 and i + 4) Cα/NH NOEs were observed (Supplementary Figure 4b, c ). Notably, long-range NOE contacts between the F2 aromatic ring protons with CαH and CβH of W7, as well as NOE contacts between the W7 NεH proton and F2 backbone and side-chain protons were observed (Supplementary Figure 4d ). In addition, the indole proton of W7 showed NOE contacts with the aliphatic side-chain proton resonances of residues I8, V11, and I12, suggesting close interactions of amino acid side-chains in LPS-bound VFR12. In summary, the analyses of tr-NOESY spectra of HVF18 and VFR12 demonstrate that LPS binding induces backbone stabilisation and (partial) formation of α-helical conformation. Structure of HVF18 and VFR12 bound to LPS micelles The 3D structure of LPS-bound HVF18 was determined from a total of 145 tr-NOE-derived distance restraints and dihedral angle restraints (Fig 4b and Table 1 ). Figure 4c superposes the backbone atoms of the 20 lowest energy structures of HVF18. The structure is well-defined, with a backbone and heavy atom RMSD of 0.88 ± 0.41 and 1.73 ± 0.46 Å, respectively. In the LPS-bound state, the C-terminus of HVF18, encompassing residues Q10-G17, forms a compact helix. In contrast, the N-terminal residues, F3-L5 are in an extended state, followed by a β-turn involving residues K6-K7-W8-I9 (Fig. 4d ). The presence of strong backbone HN/HN ( i to i + 1) NOEs, medium intensity Cα/NH ( i to i + 2), alongside the absence of Cα/NH ( i to i + 3) NOEs, confirms the formation of a type II β-turn (Fig. 4a ). Furthermore, the close proximity of the K6 carbonyl oxygen and the amide proton of I9 (2.2–2.4 Å), in all calculated structures indicate hydrogen-bond formation (Fig. 4e ). The β-turn gives the peptide backbone a curved shape with amphipathic side-chain dispositions. The side-chains of R4/K6/K7 and Q10/K11/Q15 form two hydrophilic clusters connected by the central hydrophobic W8 residue (Fig. 4f ) on the convex side; whereas, the side-chains of V2/F3/I9/V12/I13/F16 form a concave hydrophobic core (Fig. 4g ). 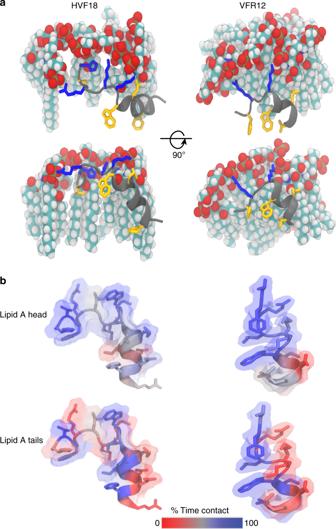Fig. 5 Molecular dynamics (MD) simulations of thrombin C-terminal peptides with lipid A aggregates.aAll-atom (AA) MD simulations of HVF18 and VFR12 showing side chains of hydrophilic (blue) and hydrophobic (yellow) residues in contact with the headgroup and lipid A acyl tail.bHVF18 and VFR12 NMR structures highlighting the side chain residue contact differences with the LPS head group and acyl chain obtained from coarse grained (CG) molecular dynamics simulations Table 1 Summary of the structural statistics for the 20 lowest energy structures of HVF18 and VFR12 in LPS micelles Full size table Likewise, the LPS-bound structure of VFR12 was determined using the tr-NOEs distance restraints (Supplementary Figure 5 and Table 1 ). The structure is well-defined with a backbone and heavy atom RMSD of 0.84 ± 0.34 and 1.70 ± 0.23 Å, respectively (Supplementary Figure 5c ). As in HVF18, the N-terminal residues (F2-L4) are extended with a β−turn (K5-I8), followed by an extremely short C-terminus helical turn I8-V11 (Supplementary Fig. 5b ). The formation of the helical segment is confirmed by the diagnostic medium-range HN/HN ( i to i + 2), Cα/NH ( i to i + 2, i + 3 and i + 4) contacts for the C-terminal residues (Supplementary Fig 5a ). Consequently, the overall structure of LPS-bound VFR12 is linear and the amphipathic distribution of side chains is disturbed. Although a hydrophilic surface, including R3/K5/K6/Q9/K10 is formed in VFR12, the hydrophobic patch is small, involving only side-chains of F2/W7/V11 (Supplementary Fig 5e, f ). 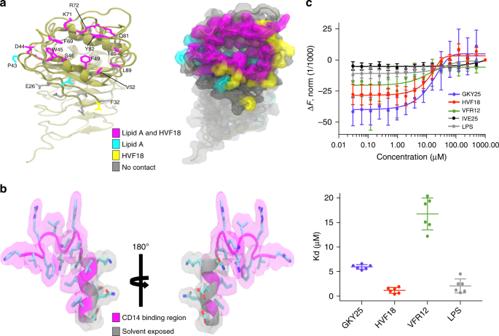Fig. 6 Thrombin C-terminal peptides interaction and binding to human CD14 ligand binding pocket.aRibbon representation of CD14 N-terminal hydrophobic pocket rim highlighting side-chains of residues contacting LPS (cyan), HVF18 (yellow), and both LPS and HVF18 (magenta) in an all-atom molecular dynamics simulation model.bRibbon representation of HVF18 indicating residues in contact with CD14 hydrophobic pocket (magenta) and solvent exposed (grey).cMicroscale thermophoresis assay quantifying CD14 interaction with TCPs and LPS. The peptide IVE25 was used as negative control. MST analysis was performed in concentration range 1000–0.03 μM of HVF18, GKY25, IVE25 and 500–0.03 μM of LPS.Kdconstants of HVF18 = 1.2 μM, GKY25 = 6.0 μM, VFR12 = 16.8 μM and LPS = 2.1 μM were determined. The results are mean values ± SD of six measurements Simulated assembly of TCPs with lipid A aggregates Next, tr-NOESY derived HVF18 and VFR12, as well as modelled GKY25, were allowed to bind (at a 1:2 ratio of peptide:lipid) to lipid A aggregates comprising 60 molecules during coarse-grained (CG) molecular dynamics (MD) simulations (Supplementary Figure 6 ). Lipid A was chosen for computational efficiency in the simulations, as it is the core effector component of LPS [15] . Divalent Ca 2+ ions included in the simulations served to crosslink phosphate moieties between lipid A molecules, and are known to be essential for the stability of the resultant lamellar phase membranes and other biologically relevant phases [24] . At t = 250 ns, large clusters of peptides were formed on the surface of the lipid aggregates. Eventually, all of these peptide clusters dispersed into the aggregate over the course of a series of ~40 μs simulations (Supplementary Figure 6a ). The positively charged N-terminal residues were observed to compete with the Ca 2+ ions that cross-linked between the phosphates of lipid A, resulting in more loosely connected headgroups (Supplementary Figure 6a ). This breaking up of the headgroup-crosslinking interactions occurred concurrently with the dispersion of the peptide clusters into the lipid aggregates. 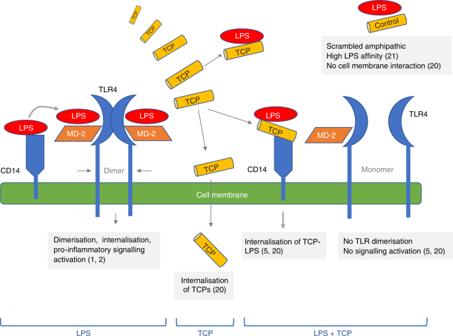Fig. 7 The multiple effects of TCPs. TCPs exert anti-inflammatory effects and protect from endotoxic shock and bacterial sepsis in experimental animal models5,7,8,22. Binding of the TCP HVF18 to LPS leads to a structural transition, wherein the peptide forms a C-shaped structure comprising a C-terminal helix, and serves in LPS scavenging and bacterial cell neutralisation. TCPs not only interact with bacteria and LPS, but also directly with monocytes/macrophages, leading to interference with TLR4 dimerization20as well as to CD14 (Kd~μM levels) on monocytes and macrophages, and may be subsequently internalised. This is proposed to competitively block CD14–LPS interaction, and/or to prevent transfer of LPS to the TLR4/MD-2 complex, thus interfering with TLR4 dimerisation and downstream inflammatory responses47. This effect is abrogated in a scrambled, amphipathic TCP sequence, which retains affinity for LPS but demonstrates no anti-endotoxic activity Once the peptides had dispersed into the lipid aggregates, the hydrophilic and positively charged residues at the N-terminus, K2, T7, H8* R11*, K13*, and K14* of GKY25 (*also in HVF18) were found to be in contact with only the head group particles of lipid A (Supplementary Figure 7 ). The aromatic residues, Y3, F5, Y6, and F10*, are interfacial residues, binding both the head and tail parts of the lipid, while the C-terminal F22* was more often in contact with the tails. The hydrophilic and negatively charged residues of the C-terminal helix were solvent exposed, and had a propensity to interact with the Ca 2+ ions after they had been displaced from their sites crosslinking lipid phosphates. Measurements of the Solvent Accessible Surface Area (SASA) of the combined peptide and lipid complexes revealed a graduated ability of the TCPs to protect the lipid A acyl tails from solvent, GKY25 providing the highest degree of protection and VFR12 the least (Supplementary Figure 6b ). Thus, the potency of LPS neutralisation may correspond directly with the peptides ability to bury the acyl tails of lipid A. Furthermore, high resolution all-atom (AA) simulations of VFR12 and HVF18 served to validate the CG simulations (Fig. 5a ). These additional simulations revealed a similar mode of binding to lipid A moieties as observed in the CG simulations, with the N-terminal positively charged residues serving to make contacts with headgroups, and the hydrophobic residues of the C-terminal helix making contacts with the lipid interfacial region and tails atoms (Fig. 5b ). Taken together, the combined CG and AA MD simulations correlate with the structural and in vitro effect studies, providing a detailed description of TCP–LPS interactions as well as regions directly contacting LPS that is reflected in the LPS neutralising capabilities of the different TCPs. Fig. 5 Molecular dynamics (MD) simulations of thrombin C-terminal peptides with lipid A aggregates. a All-atom (AA) MD simulations of HVF18 and VFR12 showing side chains of hydrophilic (blue) and hydrophobic (yellow) residues in contact with the headgroup and lipid A acyl tail. b HVF18 and VFR12 NMR structures highlighting the side chain residue contact differences with the LPS head group and acyl chain obtained from coarse grained (CG) molecular dynamics simulations Full size image LPS and TCP interaction with human CD14 CD14 is a well-known pattern recognition receptor that plays a prominent role in sensitising cells to LPS, and transferring it to the TLR4 signalling complex [25] . Considering the ability of TCPs to bind LPS and block TLR4 dimerisation at cell surfaces [5] , [20] , in silico analyses were performed to investigate possible TCP–CD14 interactions. Mutational studies suggest that charged surfaces at the amino-terminus of CD14 may be used to capture LPS and the hydrophilic rim in particular to be of importance for LPS binding and cell activation [26] . In the absence of a ligand-bound structure for CD14, unbiased all-atom MD simulations were performed with the previously reported crystal structure of human CD14 [27] , to which a nearby lipid A molecule spontaneously bound to the suggested binding cavity (Fig. 6a ). Subsequently, the energetic properties of binding a lipid A molecule to the hydrophobic pocket were investigated (Supplementary Figure 8 ) using biased all-atom MD simulations, based on an umbrella sampling (US) methodology [28] . The resultant potential of mean force (PMF) provides a measure of the lipid binding free-energy as a function of distance from the CD14 binding cavity [29] . The calculated PMF displays a smooth rise in free-energy upon extraction of lipid A from the CD14 binding cavity towards the bulk solvent phase, plateauing ~2 nm from the cavity (Supplementary Figure 8a ). The absolute free-energy change between the CD14-bound and fully solvent-dissolved states were ~200 kJ mol −1 (Supplementary Figure 8b ). This is similar in magnitude to the previously calculated binding free-energy change of lipid A to the structurally characterised LPS binding cavity of MD-2, the co-receptor of TLR4 [30] , hence confirming that the proposed N-terminal location of CD14 is indeed a true binding site for LPS molecules. Fig. 6 Thrombin C-terminal peptides interaction and binding to human CD14 ligand binding pocket. a Ribbon representation of CD14 N-terminal hydrophobic pocket rim highlighting side-chains of residues contacting LPS (cyan), HVF18 (yellow), and both LPS and HVF18 (magenta) in an all-atom molecular dynamics simulation model. b Ribbon representation of HVF18 indicating residues in contact with CD14 hydrophobic pocket (magenta) and solvent exposed (grey). c Microscale thermophoresis assay quantifying CD14 interaction with TCPs and LPS. The peptide IVE25 was used as negative control. MST analysis was performed in concentration range 1000–0.03 μM of HVF18, GKY25, IVE25 and 500–0.03 μM of LPS. K d constants of HVF18 = 1.2 μM, GKY25 = 6.0 μM, VFR12 = 16.8 μM and LPS = 2.1 μM were determined. The results are mean values ± SD of six measurements Full size image Docking of tr-NOESY derived HVF18 to human CD14 using the ClusPro server [31] indicated the peptide to be bound to the amino terminal hydrophobic pocket of CD14 in >90% of the docked models retrieved from the server (Fig. 6 ). In the majority of these structures, the N-terminal tail of HVF18 was buried deeply into the hydrophobic pocket of CD14, making clear contacts with rim residues W45, F49, V52, F69, and Y82 that bind LPS tails during simulations (Fig. 6a ). In contrast, the C-terminal helix of the peptide bound to a variety of hydrophilic rim residues, such as K71, R72, and Q81, as well as to rim residues specific for human CD14, such as the D44, S46, T85, and L89 (Fig. 6a ). In all the docked poses, HVF18 would contact CD14 in a common orientation with the C-terminal residues of Q10, K11, D14, Q15, and E18 exposed to the solvent (Fig. 6b ). In contrast, VFR12 had a less specific mode of interaction, binding to CD14 in a variety of orientations. In a few cases, VFR12 would lie across the entrance to the hydrophobic pocket, making contact with all the rim residues of CD14. A GKY25-bound state was inferred by modelling the N-terminal residues as a random coil, using HVF18 as an initial template. The highest quality models of the GKY25-CD14 complex, i.e., those with the lowest values of the objective energy function, would either loop the N-terminal residues into and out of the pocket (Supplementary Figure 9 ), or lay at the N-terminus across the entrance to the CD14 pocket, completely blocking entry. Likewise, microscale thermophoresis (MST), a highly sensitive technique probing interactions between components in solution, validated the in silico simulations presented above. As can be seen in Fig. 6c , fluorescence-labelled CD14 binds E. coli LPS, with a K d of 2.1 ± 1.4 μM, corresponding with previous reports [4] . Interestingly, both HVF18 and GKY25 showed a significant affinity to CD14 ( K d of 1.2 ± 0.6 μM and 6.0 ± 0.5 μM, respectively), contrasting the lower interaction observed for VFR12 ( K d of 16.8 ± 3.2 μM). In addition, using MST, we observed that the affinity of LPS for CD14 was significantly reduced in the presence of GKY25 and HVF18 (Supplementary Figure 10a, b ), illustrating the competitive nature of this interaction. Finally, chemical crosslinking followed by tryptic digestion and peptide analysis by tandem mass spectrometry was employed to identify the TCP-binding CD14 region. As shown in Supplementary Figure 10c , residue K14 (K 14 WIQK) of GKY25 crosslinks to K87 (QYADTVK 87 ALR) of CD14. Notably the identified sequences matched those predicted computationally (Fig. 6a ). Overall, these results indicate that the endogenous HVF18 and prototypic GKY25 efficiently block LPS-induced downstream signalling through a combination of LPS sequestration, as well as high affinity antagonistic binding to the amino terminal hydrophobic binding pocket of CD14, blocking LPS-CD14 interactions. Today, there is an increasing interest in developing HDPs as immune modulators [11] , [32] , and natural sequences such as the TCPs studied here are of interest for use in human therapy. In this perspective, it is important to define peptide actions at the molecular level for rational design and development of new peptide-based anti-infectives [33] , [34] , [35] . The current study, defining TCPs interactions with both LPS and human CD14, therefore provides a molecular and mechanistic explanation for the previously observed therapeutic effects of TCPs in experimental models of bacterial sepsis and endotoxin shock [7] , [8] (Fig. 7 for summary). Fig. 7 The multiple effects of TCPs. TCPs exert anti-inflammatory effects and protect from endotoxic shock and bacterial sepsis in experimental animal models [5] , [7] , [8] , [22] . Binding of the TCP HVF18 to LPS leads to a structural transition, wherein the peptide forms a C-shaped structure comprising a C-terminal helix, and serves in LPS scavenging and bacterial cell neutralisation. TCPs not only interact with bacteria and LPS, but also directly with monocytes/macrophages, leading to interference with TLR4 dimerization [20] as well as to CD14 ( K d ~μM levels) on monocytes and macrophages, and may be subsequently internalised. This is proposed to competitively block CD14–LPS interaction, and/or to prevent transfer of LPS to the TLR4/MD-2 complex, thus interfering with TLR4 dimerisation and downstream inflammatory responses [47] . This effect is abrogated in a scrambled, amphipathic TCP sequence, which retains affinity for LPS but demonstrates no anti-endotoxic activity Full size image Concerning the LPS-interaction, we show that the HVF18-LPS structure comprises a C-terminal helix and extended N-terminus with a β-turn (Fig. 4 ) that favours a curved backbone fold, imparting a C-shaped amphipathic arrangement of the hydrophobic core lined with two hydrophilic clusters. Over the years, tr-NOESY has been employed to obtain three-dimensional structures of LPS-interacting peptides such as lactoferrin [36] , LBP [37] , the magainin analogues MSI-78 and MSI-594 [38] , and pardaxin [39] , providing information on their mechanism of LPS-neutralisation and bacterial outer membrane permeabilisation [36] , [37] , [38] , [39] , [40] . The wide diversity of backbone folds in these structures highlights some variability among LPS-interacting structures [41] . For example, pardaxin or MSI-594 forms helix-loop-helix structures in LPS, while lactoferrin derived LF-11, LBP derived LBP-14 or a de novo designed YW12 [42] form β-hairpin or β-boomerang structures, respectively. The heparin cofactor II-derived peptide KYE28 displays an N-terminal short helical region followed by a loop, two turns, and an extended C-terminus when bound to LPS [43] . Nevertheless, a unifying feature of these determined structures is that they display partly well-defined and flexible structures in complex with LPS, characterised by an amphipathic fold. In this perspective, it is of interest that TCPs share many of these overall characteristics, although they form a unique C-shaped structure, reminiscent of the T-shaped fold of LF-11 (Supplementary Figure 11 ). The combined CG and AA molecular dynamics simulations identified key residues critical for TCPs interaction with LPS (Fig. 5 ). In contrast to HVF18 and GKY25, VFR12 lacks the N-terminal hydrophobic residues as well as the C-terminal hydrophilic residues that display increased contacts with the LPS head and acyl chain. Consequently, VFR12, though capable of still binding to LPS (via R3, K5, K6) is inefficient in caging the lipid A acyl tails from exposure to the microenvironment and thus is unable to block LPS-triggered pro-inflammatory responses. Apart from this structural information, we demonstrate a previously undisclosed interaction between TCPs and human CD14. In silico docking and MST analysis, shows that that TCPs bind with high affinity to the amino terminal hydrophobic LPS binding pocket of human CD14, the primary receptor of LPS (Fig. 6 ). Indeed, using chemical crosslinking followed by mass spectrometry analyses the crosslink site between TCP-CD14 was found to correspond to the in silico predictions for CD14 binding, identifying the TCP-sequence KKWIQK crosslinked to the LPS-binding hydrophobic pocket sequence of CD14 (QYADTVKALR) (Supplementary Figure 10 ). Interestingly, the identified TCP-region overlaps with the amino acid residues involved in the interaction with LPS (RLKKWIQK), suggesting that TCPs can interfere with LPS-CD14 interactions, hence abrogating downstream transfer of LPS to the MD-2 complex and other effectors. This is in agreement with recent simulations describing the pathway for the transfer of lipid A from CD14 to TLR4/MD2, which highlights that TCPs binding near the hydrophobic cavity could either impede the transfer of the lipid or occlude the interface between the receptor proteins (Supplementary Figure 12 ) [44] . From an evolutionary perspective, it is notable that these residues contains the cationic and aromatic amino acid residues proposed as critical for lipid A interactions [45] , present in several LPS-binding proteins [46] . It is also notable that these residues are part of the region which binds to the LPS-binding pocket of CD14, whereas the less conserved residues in the C-terminal end are outside this pocket (Supplementary Figure 13a ). In this context, it is noteworthy that a number of natural and synthetic antagonists are known to interact with CD14, acting as LPS mimics that are either delivered by CD14 or directly compete with LPS for interaction with CD14. For example, the natural antagonist lipid IVa, the natural low-toxicity partial agonist monophosphoryl lipid A, and Eritoran, a synthetic LPS antagonist structurally similar to lipid IVa, are all shuttled by CD14 to MD-2/TLR4 [47] . Further, synthetic LPS inhibitors derived from either diacylated sugars or tetraacylated sulphate–containing compounds competitively block LPS binding to CD14 [27] , [48] . Whether TCPs interact with MD-2 and TLR4, apart from CD14, remains to be investigated. However, similar to TCPs, several such inhibitors interact with the LPS-binding groove, and have been developed as potential antisepsis agents [48] , [49] . It is also notable that the TCP HVF18 [5] , [6] binds CD14 with an affinity similar to that obtained for LPS. In this context, it is therefore interesting that multiple variants of TCPs are generated by human and bacterial proteases, several of which are found in human wound fluids [6] (Supplementary Figure 13b ). This observation implies that shorter TCP fragments, related to VFR12, may be exclusively binding to LPS and bacteria, whereas longer fragments like the HVF18 or FYT21 have the capacity also to neutralise LPS and inhibit TLR4 signalling pathways. Furthermore, the fact that the major TCP fragment generated by human neutrophil elastase, HVF18, shows a higher affinity for CD14 than the longer GKY25, whereas the reciprocal applies to their interactions with LPS, illustrates that protease-mediated generation of multiple TCPs may tune LPS-responses during wounding and infection. It is also interesting that the affinities between TCPs and CD14 were in the μM range, similar to the K d of LPS to CD14. Hypothetically, this could enable TCPs to down-modulate excessive responses to bacteria and LPS responses, without completely abrogating such responses, as they also have a physiologically relevant function in infection clearance. Indeed, such phenomena have been observed in experimental models of bacterial sepsis and endotoxic shock, where treatment with TCPs reduced cytokine responses and animal mortality [7] , [8] . It has been increasingly appreciated that a multitude of weak, or transient, biological interactions ( K d >  μM), either working alone or in concert, occur frequently throughout biological systems [50] , [51] . The here disclosed TCP family, with its multiple and relatively weak affinities, all in the μM range, may represent an elegant example of such an endogenous system, with an ultimate function of modulating host responses to infection. Sharing many characteristics with transient drugs, defined by their multivalency, multiple targets, high-off-rates and K d values at μM levels [50] , TCPs could therefore be of interest in the development of novel anti-inflammatory therapies inspired by Nature. Peptides The peptides GKY25 (GKYGFYTHVFRLKKWIQKVIDQFGE), FYT21 (FYTHVFRLKKWIQKVIDQFGE), HVF18 (HVFRLKKWIQKVIDQFGE), and VFR12 (VFRLKKWIQKVI), were synthesised by Biopeptide (San Diego, CA). We confirmed the purity (over 95%) using mass spectral analysis (MALDI-TOF Voyager, USA). Digestion of α-thrombin and western blotting Human α-thrombin (4 μg) (Innovative Research, Inc, USA) was incubated with human neutrophil elastase (HNE) (Calbiochem, USA) at an enzyme-substrate ratio of 1:30 (w/w) in 10 mM Tris, pH 7.4 (volume of 10 μl) at 37 °C for 30, 60 and 180 min. After incubation, the enzyme was inactivated by heating at 95 °C for 3 min. After addition of 7 μl of Novex sample buffer and heating at 95 °C for 10 min, samples were analysed using 10–20% Novex Tricine pre-cast SDS-PAGE gel (Invitrogen, USA) run at 90 V, for 2 h. Immediately following electrophoresis, western blotting was performed at 25 V for 90 min on ice. After the transfer, PVDF membrane (Bio-Rad, USA) was blocked with 5% milk for an hour, followed by overnight incubation with rabbit polyclonal antibodies recognising the thrombin C-terminus peptide sequence (VFRLKKWIQKVIDQFGE) (Innovagen AB, Sweden) in 1:5000 dilution at 4 °C. Post washing (3 × 10 min) the membrane was incubated with HRP-conjugated goat anti-rabbit immunoglobulin G secondary antibodies (Cat no. P0448, Dako, Denmark) in 1:10,000 dilutions for an hour. Finally, the membranes was washed, TCPs were detected by SuperSignal West Pico Chemiluminescent Substrate (Thermo Fisher Scientific, USA), and visualised using a ChemiDoc MP System (Bio-Rad, USA). Fluorescence spectroscopy Fluorescence experiments were carried out with a Cary Eclipse fluorescence spectrophotometer (Varian Inc., Australia) equipped with dual monochromators using a 0.1 cm path length cuvette and a slit width of 5 nm. All fluorescence spectra were recorded in 10 mM Tris buffer, pH 7.4. Intrinsic tryptophan fluorescence spectra of free peptide were recorded using 5 μM peptide and the interaction with LPS was studied by titrating the peptide with increasing lipid concentration up to 10 μM. The intrinsic tryptophan was excited at a wavelength of 280 nm and the emission monitored between 300 and 400 nm. The change in emission maxima was used to determine the LPS binding affinity of the peptides using Graph Pad Prism v7.02 (GraphPad Software, Inc. USA), assuming a single binding site. Acrylamide (stock 5 M) was used to quench the fluorescence of the tryptophan residue. Increasing concentrations of acrylamide was added stock 5 M into 10 mM Tris buffer, pH 7.4, containing either unbound (5 μM) peptide or in the bound state containing saturating concentration of LPS (10 μM). Spectra shown are representative of three experiments. Quenching of fluorescence intensity at emission maxima for corresponding free and lipid-bound forms was analysed using the Stern-Volmer equation, 
    F_0/F = 1 + K_sv[ Q],
 (1) where F o and F are the fluorescence intensity at emission maxima in the absence and presence of quencher, respectively, K SV is the Stern-Volmer quenching constant, and [Q] is the molar concentration of quencher [50] . Results shown are means ± standard deviation (SD) of three experiments. Ellipsometry Peptide adsorption was studied in situ by null ellipsometry [52] , using an Optrel Multiskop (Optrel, Kleinmachnow, Germany) equipped with a 100 mW Nd:YAG laser (JDS Uniphase, Milpitas, USA). All measurements were carried out at 532 nm and an angle of incidence of 67.66° in a 5 ml cuvette with stirring (300 rpm). In brief, by monitoring the change in the state of polarisation of light reflected at a surface in the absence and presence of an adsorbed layer, the mean refractive index ( n ) and layer thickness ( d ) of the adsorbed layer can be obtained. From the thickness and refractive index, the adsorbed amount ( Γ ) was calculated according to: 
    Γ = ( n - n_0)/dn/dcd,
 (2) where d n /d c (0.154 cm 3 g −1 ) is the refractive index increment and n 0 is the refractive index of the bulk solution. Corrections were routinely done for changes in bulk refractive index caused by changes in temperature and excess electrolyte concentration. LPS-coated surfaces were obtained by adsorbing E. coli LPS to methylated silica surfaces (surface potential −40 mV, and contact angle 90°) from 5 mg ml −1 LPS stock solution in water at a concentration of 0.4 mg ml −1 in 10 mM Tris, pH 7.4. This LPS concentration corresponds to saturation in the LPS adsorption isotherm under these conditions. Non-adsorbed LPS was removed by rinsing with Tris buffer at 5 ml min −1 for a period of 30 min, allowing the buffer to stabilise for 20 min. Peptide addition was subsequently performed to 0.01, 0.1, 0.5, and 1 µM, and adsorption monitored for at least 1 h after each addition. Data shown are means ± SD of two experiments performed in duplicates at 25 °C. Limulus amebocyte lysate (LAL) assay The ability of peptides to sequester LPS was assayed using a commercially available LAL chromogenic kit (QCL100 Cambrex, Lonza, USA), according to the manufacturer’s protocol. LPS activates a proenzyme in the Limulus amebocyte lysate (LAL), which in turn catalytically splits a colourless substrate to the coloured product para-nitroanilide (pNA), which is measured spectrophotometrically at 410 nm. Data shown are mean values ± SD of two experiments. Prior to running the assay, the peptides were dissolved at 200 μM in pyrogen-free water, supplied with the kit. NF-κB activation assay THP1-XBlue-CD14 reporter cells (1 × 10 6 cells ml −1 ) (InvivoGen, San Diego, USA) were seeded in phenol red RPMI (180,000 cells/well), supplemented with 10% (v/v) heat-inactivated FBS and 1% (v/v) Antibiotic-Antimycotic solution (AAS), and allowed to adhere before they were stimulated with 100 ng ml −1 LPS ( Escherichia coli serotype 0111:B4) (Sigma, USA) and with peptides at the indicated concentrations. The NF-κB activation was determined after 20 h of incubation according to the manufacturer’s instructions (InvivoGen, San Diego, USA). Briefly, activation of NF-κB leads to the secretion of embryonic alkaline phosphatase (SEAP) into the cell supernatant, where it is measured by mixing the supernatant with a SEAP detection reagent (Quanti-Blue TM , InvivoGen), followed by absorbance measurement at 600 nm. Data shown are mean values ± SD obtained from at least six experiments. CD spectroscopy The secondary structure of unbound and LPS-bound peptides was analysed by circular dichroism (CD) spectroscopy using a Chirascan Circular Dichroism spectrometer, (Applied Photophysics, UK) with a cuvette of path length of 0.05 cm (Hellma, GmbH & Co, Germany). Spectral data were collected at a step size of 0.5 nm, time constant of 1 s and peptide concentration of 20 μM in 10 mM Tris, pH 7.4. Structural changes upon addition of E. coli 0111:B4 LPS (100 μM), was recorded in the same buffer. The molecular weight of LPS was considered to be 10 kDa, according to a previous report [53] . All spectra were recorded at 25 °C from 190 to 260 nm, using a bandwidth of 1-nm, and averaged over three scans. Baseline scans were obtained using the same parameters for buffer or LPS and subtracted from the respective data scans with peptides. The final corrected averaged spectra were expressed in mean residue ellipticity. NMR spectroscopy All NMR experiments were performed on a Bruker DRX 600 MHz spectrometer (Bruker, Germany), equipped with cryo-probe and pulse field gradients. NMR data processing and analysis was carried out using Topspin software (Bruker) and the SPARKY NMR assignment program ( https://www.cgl.ucsf.edu /home/sparky). Two-dimensional 1 H– 1 H TOCSY and 1 H– 1 H NOESY spectra of GKY25, FYT21, HVF18, and VFR12 were acquired at 298 K at a peptide concentration of 0.5 mM in aqueous solutions containing 10% D 2 O, pH 4.5 at a mixing time of 80 and 200 ms, respectively. 4,4-dimethyl-4-silapentane-5-sulfonate sodium salt (DSS) was used as an internal standard (0.0 ppm) in all NMR experiments. The peptide-LPS interaction was monitored by a series of one dimensional 1 H-NMR spectra titrated with various concentrations of LPS until line broadening was observed. Two-dimensional tr-NOESY experiments for VFR12 and HVF18 were acquired in the presence of 20 μM and 30 μM LPS with mixing times of 100, 150 and 200 ms. The peptide-LPS complex was stable over the period of data collection and generated a large number of tr-NOE cross-peaks. All two-dimensional tr-NOESY experiments were performed with 400 increments in t1 and 2048 data points in t2 using WATERGATE [54] procedure for water suppression and States-TPPI [55] for quadrature detection in the t1 dimension. The spectral width was 12 ppm in both dimensions. After 16 dummy scans, 80 scans were recorded per t1 increment. After zero filling in t1, 4 K (t2) × 1 K (t1) data matrices were obtained. Motivated by previously reported preferential binding of TCP to LPS over lipid membranes [21] , [56] , as well as the focus on LPS interactions in the present investigation, LPS micelles were chosen for these studies. It should be noted, however, that TCPs adopt similar conformation in other frequently used membrane-mimetic systems, indicating peptide conformation to depend relatively weakly on curvature and membrane headgroup (Supplementary Figure 14 ). Having said that, the atomic resolution structures of peptides may change in detergent micelles, as reported recently by Chipot et al. [57] . Therefore, although outside the scope of the present study on LPS/CD14-interactions, the broader issue of impact of composition and structure of membrane-mimetic systems on the conformation of TCPs needs to be followed up in future investigations. NMR-derived structure calculations The LPS-bound three-dimensional structures of VFR12 and HVF18 were calculated using the CYANA program (version 2.1) [58] from tr-NOESY (mixing time 150 ms) derived distance constraints. NOE intensities were qualitatively assigned to strong, medium, and weak cross-peak intensities with upper bound distance limits of 3.0, 4.0, and 5.5 Å, respectively. The lower bounds for all distance restraints were fixed to 2.0 Å. The backbone dihedral angle (Phi) was varied between −20° and −180° to reduce conformational sampling. No hydrogen bond constraints were used for structure calculation. Several rounds of structure calculations were performed and depending on the NOE violations, the angle and distance constraints were refined. Finally, out of 100 generated structures, the 20 lowest energy conformers with low RMSD were selected for the NMR ensemble. Structures were visualised using the MOLMOL and PyMOL software. The quality of the determined structure was validated using PROCHECK-NMR [59] . Peptide assembly simulations to LPS aggregates All molecular dynamics (MD) simulations were performed using the GROMACS simulation package [60] . All-atom (AA) MD simulations of VFR12 and HVF18 were performed using the CHARMM27 force field including additional CMAP potentials [61] . Electrostatic interactions were treated using the smooth Particle Mesh Ewald (PME) method [62] , with a cutoff for short-range interactions of 1.2 nm. The van der Waals interactions were switched to zero between 1.0 nm and 1.2 nm. The system temperature was maintained at a constant temperature of 313 K using the velocity-rescale thermostat and a coupling constant of 1 ps [63] . A pressure of 1-bar was maintained isotropically using the Parrinello-Rahman barostat and a coupling constant of 5 ps. To ensure that the conformational space accurately reproduced the tr-NOESY derived structures, the NOEs were modelled in the simulations as flat-bottomed distance restraint potentials with a force constant of 1000 kJ mol −1 nm −2 . The time constant for the distance restraints running average was 10 ns. Angle restraints of 100 kJ mol −1 rad −2 were also applied to maintain the experimentally-derived backbone conformation. A lipid A aggregate was created by manually positioning ten lipid A molecules in solution using VMD [64] and allowing them to self-assemble over a timescale of 100 ns. The lipid parameters were developed using CHARMM27 building blocks [47] . The peptides were positioned ~2.0 nm from the aggregate surface. Energy minimisation, using the steepest descent algorithm, was performed for 1000 steps. Position restraints, with a force constant of 1000 kJ mol −1 nm −2 , were placed on the Cα particles of the peptides for 5 ns. Production simulations were performed for 250 ns. CG MD simulations were performed using the MARTINI 2.2 force field [65] . DSSP was used to determine the secondary structures of the tr-NOESY derived VFR12 and HVF18 structures. The DSSP secondary structure categories served as constraints in the preparation of MARTINI protein parameters [66] . The additional seven residues at the N-terminus of GKY25, with respect to HVF18, were modelled as a random coil. The MARTINI protein parameters were optimised to reproduce the average ensemble properties of the atomistic simulations. Details of the optimisation procedure are provided in Supplementary Method. The large lipid A aggregate was created by allowing 60 randomly placed lipid molecules to assemble over the course of a 1 μs simulation. The final frame of this simulation was used as the starting point for the creation of three further systems in which 30 GKY25, HVF18 or VFR12 peptides, respectively, were scattered randomly in the simulation cell, all at least 2 nm from the aggregate. The GKY25, HVF18, and VFR12 CG production simulations were each run for 10 μs. A simulation of the aggregate alone, with no peptides added, was also extended to 11 μs, and this served as negative control. All CG simulations were maintained at a constant temperature of 313 K using velocity rescale thermostat [63] . A system pressure of 1 bar was maintained isotropically using the Parrinello-Rahman barostat [67] , [68] with a coupling constant of 20 ps. Electrostatic interactions were treated using the reaction-field method [69] with a dielectric constant of 15 within a 1.1 nm cutoff, and zero beyond the cutoff. The van der Waals interactions were shifted to zero at 1.1 nm. Peptide and LPS interference with CD14 interactions The tr-NOESY derived structures of VFR12 and HVF18 were docked to human CD14 using the ClusPro server [31] . The structure of CD14 with GKY25 bound was modelled using Modeller v9.15 [70] with the HVF18-CD14 complex model as a template via the loopmodel function with the MD refinement set to refine.very_slow. A total of 100 models of the GKY25-CD14 complex were generated. The structure with the lowest value of Modeller’s objective function was selected for visualisation in Fig. 6 . In order to validate the GKY25-CD14 model, GKY25 was also modelled in isolation using tr-NOESY derived structure of HVF18 as a template. One hundred models were generated, and the model with the lowest objective function was selected for further docking studies. The modelled GKY25 structure was docked to human CD14 using the ClusPro server. Lipid A was assembled in an unbiased mode to CD14 via molecular simulations. Initially, a single lipid A molecule was placed ~2.0 nm from the binding pocket (measured from the center of mass of the terminal acyl carbons of lipid A to the center of the cavity). Rapid spontaneous adsorption and insertion of lipid A into the CD14 N-terminal binding cavity was observed (within 10 ns). The simulation was subsequently run for over 1 μs and the lipid molecule remained stably bound within the N-terminal pocket. For free-energy calculations, the lipid A bound CD14 structure was extracted after 1 μs of simulation. The protein and ligand were manually positioned so that pulling the lipid A molecule along the unit cell z -axis would correspond to the axis of the cavity mouth. The system was then re-solvated and minimised before a 4 ns steered MD simulation was performed, pulling the lipid A molecule 4 nm from the protein using a pulling force of 1000 kJ mol −1 nm −2 . Forty windows were extracted at 0.1 nm intervals from this trajectory for subsequent umbrella sampling (US). During US, each window was sampled for 50 ns. The lipid A sugar backbone and phosphate groups served as the reference point of the ligand, and the backbone atoms of residues 8–12 and 31–35 corresponding to the first two LRRs at the cavity entrance, were used as the reference point for CD14. Microscale thermophoresis (MST) MST analysis was performed using a NanoTemper Monolith NT.115 apparatus (Nano Temper Technologies, Germany). A Monolith NT Protein labelling kit RED – NHS (Nano Temper Technologies, Germany) was used to label 3 μM of sCD14 (PeproTech, USA) according to the manufacturer’s protocol. A constant amount of 0.5 μM of sCD14 was incubated for 30 min at room temperature with increasing concentrations of VFR12, HVF18, GKY25 (1000–0.03 μM) or LPS (500–0.03 μM) in Tris buffer (10 mM, pH 7.4). Next, 10 μl of the sample was loaded into standard glass capillaries (Monolith NT Capillaries, Nano Temper Technologies), and the MST analysis was performed (settings for the light-emitting diode and infrared laser were 80%). Labelled IVE25 was added to sCD14 under the same conditions as above and used as negative control. Similarly, for the CD14–LPS interactions in the presence of TCPs, the samples contained 3 μM of labelled sCD14 and 3 μM of TCPs or IVE25, pre-incubated in the dark at room temperature for 30 min. Then, MST analyses were performed with increasing concentration of LPS (0.03–500 μM). Results shown are mean values ± SD of six measurements. Chemical cross-linking and mass spectrometry analysis Chemical crosslinking using BS3, a water soluble homobifunctional crosslinker, was performed according to instructions from the manufacturer (Thermo Scientific, USA). Briefly 30 μM of sCD14 (PeproTech, USA) was mixed together with 30 μM of GKY25 in endotoxin-free water (G-Biosciences, USA) in total volume 30 μl. Freshly made SB3 (Thermo Scientific, USA) was added to the mixture to the final concentration 150 μM. The samples were incubated on ice for 2 h and the reaction was quenched by adding 1 M Tris to a final concentration of 50 mM. A total of 200 mM DTT was added to a final concentration 10 mM to the sample and heated at 56 °C for 30 min. A total of 200 mM iodoacetamide was subsequently added to a 50 mM final concentration, and incubation performed at room temperature in the dark for 45 min. Precipitation of proteins was performed by adding 4× volume of ice cold acetone and incubation at −20 °C overnight. In solution digestion of cross-linked proteins was done in 50 mM ammonium bicarbonate pH 8 with trypsin (1:50, w-w) overnight at 37 °C. Acidification was done by adding formic acid prior to injection of samples for LC–MS/MS. LC–MS/MS analyses were performed on an Orbitrap Fusion Tribrid Mass Spectrometer (Thermo Scientific, USA) equipped with an Easy-nLC 1000 Liquid Chromatograph (Thermo Scientific, USA). For LC separation, the mobile phases were solvent A (0.1% v/v formic acid in LC–MS grade water) and solvent B (0.1% v/v formic acid in acetonitrile). Peptides were loaded onto the trap column, an Acclaim PepMap C18 column (3 µm particle size, with an inner diameter of 75 µm and a length of 20 mm) (Thermo Scientific, USA). Next, gradient elution was performed on an Acclaim PepMap C18 column (100 Å, 3 µm, 250 mm, 75 µm). During this elution step, the proportion of solvent B increased from 1 to 30% in the first 50 min, then to 60% over 15 min, then to 90% over 5 min, and thereafter maintained for the next 5 min at a constant flow of 300 nl/min. A Proxeon nanospray source equipped with a 40 mm stainless steel emitter, a spray voltage of 1.9 kV, and capillary temperature at 275 °C was used. Data acquisition was performed using a top N method with 3 s cycle time. In MS 350–1350 m/z was scanned at a resolution of 120,000 FWHM. Selected precursors were fragmented with Orbitrap CID-MS2 with a collision energy of 35% at a resolution of 15,000 FWHM resolution using a 1.6 m/z window. BS3-cross-linked peptides were identified with the software StavroX version 3.6.6.6 with the following settings: Trypsin was chosen as the enzyme, with one missed cleavage allowance. Oxidation of methionine was treated as dynamic modifications while carbamidomethylation of cysteine was treated as fixed. Per peptide, the maximum number of post-translational modifications was 2. MS mass tolerance 5 ppm, MS/MS mass tolerance 6 ppm, up to two missed cleavages for trypsin. Data availability Data supporting the findings of this manuscript are available from the corresponding author upon reasonable request. The atomic coordinates and NMR constraints of LPS-bound HVF18 and VFR12, energy minimised conformers, are deposited in Protein data bank (PDB) with the accession codes 5Z5X and 5Z5W respectively.